Bright e-Paper by transport of ink through a white electrofluidic imaging film Many of the highest performance approaches for electronic paper use voltage to reveal or hide dark pigments or dyes over a white pixel surface, and the reflectance of white pixels is lower than in real paper because the dark pigments or dyes can never be fully removed from the visible pixel area. Here, we introduce a re-designed approach for electronic paper that transposes coloured ink in front of or behind a white microfluidic film. Pixels can provide >90% reflective area and have demonstrated <15 ms switching for 150 pixels-per-inch resolution. This new approach is also the first of its kind for electrowetting-style displays by allowing non-aligned lamination fabrication, and is the first ever colourant-transposing pixel that eliminates the need for ink microencapsulation or pixel borders. Many consumers are not aware that electronic displays significantly compromise the potential capability for portable electronic devices and electronic signage. For example transmissive LCD and emissive OLED displays themselves are thin, but they require significant power causing the battery to often become the single heaviest component in a mobile device. These same displays that provide brilliant colour indoors, collapse in colour and contrast in sunlight down to levels far below even common newsprint [1] . Furthermore, LCD and OLED suffer from an unavoidable compromise between portability and screen size. Electronic paper (e-Paper) technology like E-Ink can in theory resolve all three shortcomings by holding an image without electrical power, using reflected sunlight to create the screen image and more easily allowing rolling/folding compaction of the screen size [2] , [3] . However, e-Paper is far from universal in usage, because there is a lack of a single technology that can provide both colour reflection greater than R ∼ 20% and image updates fast enough for at least crude video [1] . Furthermore, even in monochrome operation, no e-Paper technology has yet reproduced the quality of magazine print with R =3% black/ R =76% white. We report here a completely redesigned approach for e-Paper, we refer to as an ‘electrofluidic imaging film’. Unique from the dozen or more existing e-Paper technologies [1] , an ink is electromechanically transported to the viewable front, or hidden in the back, of a highly engineered porous film. This film is a first for all types of electrowetting-style displays by allowing non-aligned lamination fabrication [3] , [4] , [5] . Furthermore, the film is able to efficiently split merged fluid and therefore eliminate the need for ink microencapsulation [6] , [7] , [8] or pixel borders needed in other displays that also move a colourant [2] , [3] , [5] , [5] . We have designed and fabricated 25 and 150 pixels-per-inch (PPI) versions of this electrofluidic imaging film. We demonstrate the operation of these films and discuss pixel aliasing, grayscale generation and calculated optical performance for both monochrome and colour e-Paper. Cumulatively, these advances provide an electrofluidic imaging film that has fast switching (<15 ms), potential for exceeding magazine quality reflectance ( R >76%) and simpler manufacturing by non-aligned lamination. Although this work represents only initial proof of concept, longer term development could advance both performance and affordability for e-Readers, smartphones/tablets and signage. Device design and theory The overall goal of this work was to create a paper-like display by using a white porous film through which immiscible black (ink) and clear (oil) fluids can be electrically transported ( Fig. 1 ). The ink transport is driven by an electromechanical pressure that counteracts the Laplace pressure that is geometrically imparted on the ink by its surroundings [4] . The Laplace pressure is calculated as Δ P = γ (1/R H + 1/R V ) where R H and R V are the horizontal and vertical radii of curvature of the ink meniscus, and γ is the interfacial surface tension between the ink and the oil. By using upper and lower channels ( Fig. 1 ) with equal thickness, h , which are hydrophobic such that R V =h/2 and have a value of h such that R V <<R h , the Laplace pressure for the ink in both the upper and lower channel can be approximated as ΔP=2γ/h. 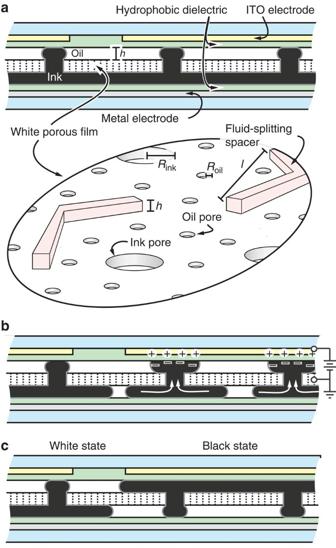Figure 1: Illustration of device structure and operation. (a) Side view of the electrofluidic imaging film in its static off state with ink stable in the hidden (lower) channel. Additional important features are shown in the angled view diagram of the white film (lower panel). The white porous film is coated with a thin reflective electrode and spacers are also present on the opposite side of the film (not shown, see Methods section). (b) Side view after voltage has been applied to one of the top electrodes and (c) after ink has merged in the visible channel and voltage is removed. Figure 1: Illustration of device structure and operation. ( a ) Side view of the electrofluidic imaging film in its static off state with ink stable in the hidden (lower) channel. Additional important features are shown in the angled view diagram of the white film (lower panel). The white porous film is coated with a thin reflective electrode and spacers are also present on the opposite side of the film (not shown, see Methods section). ( b ) Side view after voltage has been applied to one of the top electrodes and ( c ) after ink has merged in the visible channel and voltage is removed. Full size image To achieve movement, electromechanical pressure locally reduces the pressure as predicted [4] by ΔP=−CV 2 /h , where C is the capacitance of the hydrophobic dielectric and V is the voltage applied to the electrode towards which the ink will move [5] , [9] . The minimum V for movement can be very low, but practically ranges from 5 to 30 V depending on C and/or the required switching speed. Over similar distances, the speed of ink transport is ∼ 100 × faster than the conventional electrophoretic approach [4] , [7] . The faster speeds up to ∼ 10–20 cm s −1 are achieved for two reasons. First, coloured pigment particles are moved with the ink fluid not through the ink fluid (drag force), and second, the electrical field driving the ink is localized to the meniscus of the ink and does not drop across the entire length of the transport path. All of the novel features for this work directly stem from the unique and sophisticated fluid mechanics of the porous white film. Several iterative cycles of theory and experiment identified that fundamentally, the film must satisfy several key principles. First, it must be able to transport both ink and oil. Second, it must ensure a portion of the ink is always in a position such that it can receive electromechanical force from an electrode. Third, it must work without the need for alignment to electrodes. Finally, it must allow the merged ink in either channel to be locally split for rapid removal from that channel. The first three requirements are solved by ink and oil pore design, whereas the final requirement is solved by the spacers ( Fig. 1a , angled view diagram). First, the impact of the pores design is discussed. If the transport is to be efficient, there must be pores dedicated only for oil transport and only for ink transport. Because the film is hydrophobic, the pore radius R pore can be used to impart Laplace pressure that determines which fluid type fills each pore type. The pores are cylinders such that the Laplace pressure for the ink in a pore is ΔP =2 γ/R pore , because R H = R V = R pore . If the pores are made small, the Laplace pressure in the pore is larger than in the channel and ink will never fill the pore therefore creating an oil pore ( R oil <h) . Conversely, if the Laplace pressure in the pore is smaller than in the channel, ink will always fill this ink pore and rest against the top or bottom hydrophobic dielectric ( R ink >h) . More practically, due to expected fabrication variations one would further decrease/increase the targeted oil/ink pores radii by 10% or more, respectively. The density of pores is important for several factors: switching speed (more pores=less distance to travel); reflectivity (less pores=higher reflective area); and pixel resolution (at least several pores are needed per pixel electrode such that the film can be laminated without alignment to the electrodes). Second, the critically important role of the spacers is discussed, which is far beyond the purpose of conventional pixel spacers or borders [1] . The spacers provide a new method of splitting a volume of fluid from within, a capability not previously demonstrated in electrowetting or electrofluidics. Consider the conceptual scenario of the oil splitting a sheet of ink in a channel without spacers. As the oil would begin to split the ink, it would form a very small cylinder of oil surrounded by the ink. At the onset of this conceptual splitting, the oil would have a negative R H approaching zero, and therefore a near infinite ΔP , causing the pocket of oil to collapse. The spacers solve this problem by providing a stable starting condition for R H that reduces the required pressure difference between channels for splitting the ink, effectively lowering the energy barrier between merged and split ink states. The time-resolved evolution of ink splitting at a spacer is shown in Fig. 2a . The threshold ΔP for ink splitting is easy to calculate. With reference to the ink transition from Fig. 1a and b , and the ink splitting shown in Fig. 2 , assume voltage drives the ink to the top channel at ∼ ½ the maximum available pressure ΔP = CV 2 /h=γ/h . If merged ink surrounding a spacer in the lower channel is to dewet from the spacer, the spacer must lower the pressure by at least that same ΔP= γ/h. For a spacer with an end-to-end length l ( Figs 1a and 2b ), as ink dewets from a spacer, a minimally negative horizontal radius of curvature appears at the threshold pressure for splitting ( R H =−l/ 2). Therefore, equating this threshold pressure for splitting with the electrically applied pressure in the other channel, it is determined that the spacer must be designed such that l>2h . By allowing the ink to freely merge or split in either channel, these specialized spacers also completely eliminate the need for ink microencapsulation [6] , [7] , [8] or pixel borders, a novelty compared to all previous pixel approaches that move a colourant [2] , [3] , [4] , [5] . The spacers can be straight or, as shown in this work, slightly bowed between 120 and 140° for an R H that is initially slightly positive to provide a small starting volume of oil. An added effect of this bowing is a predictable direction of oil expansion experimentally shown and diagrammed in Fig. 2b . 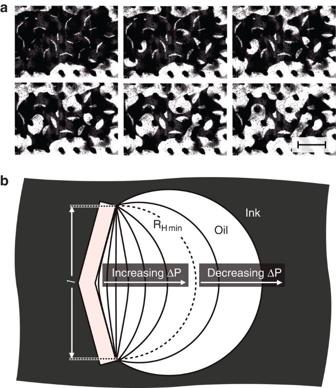Figure 2: The evolution of oil/ink interface near a splitting feature during switching. (a) Time stepped captures of splitting process showing expansion of the oil from initial stable state to 15 ms in 3 ms time intervals. Dark area is pigment and clear area is oil. Scale bar, 1 mm. (b) An illustration of the interface evolution for a single spacer. Figure 2: The evolution of oil/ink interface near a splitting feature during switching. ( a ) Time stepped captures of splitting process showing expansion of the oil from initial stable state to 15 ms in 3 ms time intervals. Dark area is pigment and clear area is oil. Scale bar, 1 mm. ( b ) An illustration of the interface evolution for a single spacer. Full size image This completes the theoretical design and operation of the electrofluidic film. Readers interested in additional details on the electromechanical pressure (electrowetting) control are encouraged to read previous work on electrofluidic displays [4] , [5] . Demonstration and characterization Devices were fabricated at two resolutions, 25 PPI ( h =50 μm, R ink =50 μm, R oil =10 μm) and 150 PPI ( h =8 μm, R ink =8 μm, R oil =1 μm). For an electrofluidic film, PPI is defined as the pixel pitch being at least twice the ink pore spacing, such that each pixel has multiple ink pores regardless of how the film is aligned to the electrodes. Presented in Fig. 3 are switching photographs for a 25 PPI film ( Fig. 3a ) using a red ink on white electrofluidic imaging film ( Fig. 3b ). It can be seen that the segments of the numeric display are approximately 2 pixels in width such that the edges of the pattern look rough in the stable state. At the appropriate viewing distance, this roughness is visually interpolated as a soft edge (below the viewers threshold of perception). Also as shown, the high-speed photographs confirm that the desired fluid break-up is achieved during switching. Using the 10 to 90% criteria described in the Methods section, the switching speed of 25 PPI device was measured to be 30 ms ( Fig. 5a ), which is fast compared with the electrowetting and previous electrofluidic approaches that become much slower at <25 PPI pixel resolutions. When voltage was removed from the device in a stable state, only 1% change in reflective area was measured. Constant stability was observed up to several hours without any measureable change. This reduces electrical power required for operation, an important advantage for e-Paper applications. Lastly, it is noted that actuation of ink in one area of the device had no observable effect on ink in other areas of the device despite the ink being interconnected, suggesting benefit from viscous drag forces and wetting hysteresis. 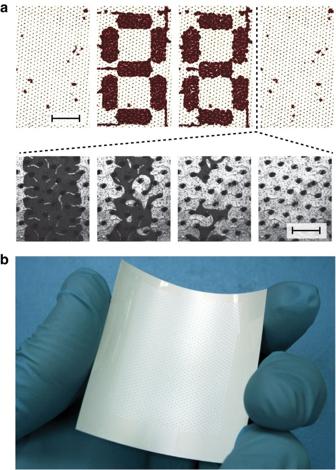Figure 3: Demonstration of a 25 PPI device. (a) Snapshots of device in four states: pigment hidden, voltage off; pigment displayed, front voltage on; pigment displayed, voltage off; pigment hidden, back voltage on. Between state 3 and 4, the lower panels show zoom-in photos of ink splitting similar to those shown inFig. 2abut showing switch to completion and at 10 ms intervals. Dark area is pigment and clear area is oil. Scale bars, 4 and 1 mm respectively. (b) Photograph of a 25 PPI film outside of the device. Figure 3: Demonstration of a 25 PPI device. ( a ) Snapshots of device in four states: pigment hidden, voltage off; pigment displayed, front voltage on; pigment displayed, voltage off; pigment hidden, back voltage on. Between state 3 and 4, the lower panels show zoom-in photos of ink splitting similar to those shown in Fig. 2a but showing switch to completion and at 10 ms intervals. Dark area is pigment and clear area is oil. Scale bars, 4 and 1 mm respectively. ( b ) Photograph of a 25 PPI film outside of the device. Full size image Figure 5: Measured performance of 25 and 150 PPI devices. 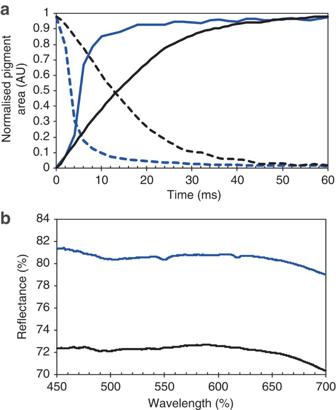Figure 5: Measured performance of 25 and 150 PPI devices. Plots of (a) devices switching speed. Black lines are results for 25 PPI devices, and blue lines are results for 150 PPI devices. Dashed lines are the change in pigment coverage as pigment is pulled to the bottom channel (white state). Solid lines are the responses as the pigment is pulled to the top channel (dark state). (b) Measured specular-included reflectance for 150 PPI films. Blue line is the reflection of the film outside of the device. Black line is the reflection of the assembled device in the white state. Plots of ( a ) devices switching speed. Black lines are results for 25 PPI devices, and blue lines are results for 150 PPI devices. Dashed lines are the change in pigment coverage as pigment is pulled to the bottom channel (white state). Solid lines are the responses as the pigment is pulled to the top channel (dark state). ( b ) Measured specular-included reflectance for 150 PPI films. Blue line is the reflection of the film outside of the device. Black line is the reflection of the assembled device in the white state. 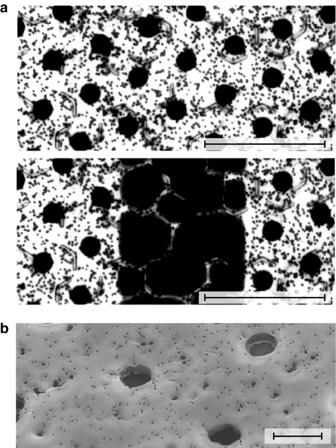Full size image By scaling all the dimensions of the film, the resolution can be increased such that a sharper image can be obtained. Figure 4: Demonstration of a 150 PPI device. (a) Bright-field photos of operation with a transparent∼200 μm wide ITO electrode and 150 PPI film. Dark area is pigment and clear area is oil. Scale bar, 200 μm. (b) SEM close up of the ink and oil pores. Scale bar, 25 μm. It should be noted that the bright-field and SEM photographs cause light-scattering features to look darker than they do at a distance to the naked eye. Figure 4 shows a 150 PPI device switching a 200-μm electrode line. An added advantage of scaling to smaller dimensions is that it leads to a decrease in switching time [9] . Accordingly, both 25 and 150 PPI device switching profiles are plotted in Fig. 5a . The switching times for 150 PPI devices were measured at <15 ms for on and off, which qualifies the pixel as achieving video rate switching speed. It should be noted that an asymmetry was observed in the switching of the 150 PPI device, which is likely attributable to channel variance that is more easily controlled in the low-resolution device. This can also lead to varying levels of stability for 150 PPI devices, suggesting the need for more repeatable fabrication/assembly. Figure 4: Demonstration of a 150 PPI device. ( a ) Bright-field photos of operation with a transparent ∼ 200 μm wide ITO electrode and 150 PPI film. Dark area is pigment and clear area is oil. Scale bar, 200 μm. ( b ) SEM close up of the ink and oil pores. Scale bar, 25 μm. It should be noted that the bright-field and SEM photographs cause light-scattering features to look darker than they do at a distance to the naked eye. Full size image Using the standard outlined in the Methods section, the reflectance of the film alone was measured at 80% ( Fig. 4b ). When the membrane was integrated into a device, a 10% loss was seen due to thin-film losses and inefficient light outcoupling [10] . The resulting white state reflectivity for the full device was found to be 72%. This is very high white reflectance, especially when compared with other pixel approaches that can switch at video speed [1] . Dark state and contrast ratio will be provided in the Discussion section. Although the achieved experimental results are preliminary, they are already quite promising in performance. Furthermore, the experimental results confirmed the theoretically expected operating principles. The first topic of discussion is related to alignment of electrodes, spacers and features of the film. To keep film fabrication simple, the pores and spacers are not aligned to each other during fabrication. However, this can cause aliasing due to periodic arrangement of features that is objectionable in terms of fluid mechanics and visual appearance. The periodic alignment of splitting spacers and ink pores can cause large dead areas, where spacers repeatedly overlap and block ink pores and\or result in visual patterns easily detected by the human eye. A similar visual issue that was observed for in-plane electrophoretic displays which displayed diffraction effects at regular arrangements of features but was resolved using randomized Voronoi patterns [11] . For this electrofluidic film, a custom computer programme was written to auto generate mask patterns for the various features of the device, and a variable amount of noise was inserted into the locations of the spacers. 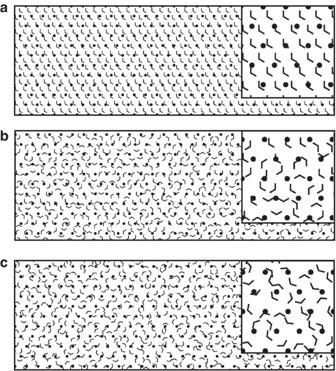Figure 6: Designs of splitting spacers with computationally increased noise and therefore a decrease of aliasing effects. Bent lines are splitting spacers. Filled circles are pigment pores. Oil pores are not shown. (a) A device design with a regular hexagonal lattice of splitting spacers with no added noise resulting in large contiguous areas of blocked pores. (b) A device design with a moderate amount of noise added in both the lattice offset and rotation such that no contiguous areas of blocked pores or clustering of spacers are observed. (c) A device design with a high amount of noise such that no contiguous areas of pore blocking are observed, but clustering of spacers is observed. Zoom-in views of the patterns are provided in the respective panel insets. Figure 6 shows three patterns generated by the programme, each with increasing levels of noise making it more difficult to detect patterns in the alignment. However, an over application of noise, as in Fig. 6c , can lead to undesirable clumping of spacers. Figure 6: Designs of splitting spacers with computationally increased noise and therefore a decrease of aliasing effects. Bent lines are splitting spacers. Filled circles are pigment pores. Oil pores are not shown. ( a ) A device design with a regular hexagonal lattice of splitting spacers with no added noise resulting in large contiguous areas of blocked pores. ( b ) A device design with a moderate amount of noise added in both the lattice offset and rotation such that no contiguous areas of blocked pores or clustering of spacers are observed. ( c ) A device design with a high amount of noise such that no contiguous areas of pore blocking are observed, but clustering of spacers is observed. Zoom-in views of the patterns are provided in the respective panel insets. Full size image The second point of discussion relates to grayscale generation. Grayscale was not characterized in this preliminary work, but simple experiments showed achievable intermediate reflectance (grayscale) using pulse-width modulation [1] , [5] . In theory, analogue control ( Q = CV ) is also possible. Bit-depth for grayscale has not yet been determined. For high-quality grayscale with pulse-width modulation, one will likely need to either introduce sufficient wetting hysteresis to improve stability of intermediate positions of the ink and/or overshoot (increase) the pixel resolution to increase the number of ink pores per pixel, thereby reducing pixel-to-pixel speed variation. For analogue control, such overshooting of resolution is not needed. Some applications such as electronic signage, require no grayscale control. The third point of discussion relates to optimized reflectivity and comparison to existing technologies. The electrofluidic imaging film of this work is able to efficiently hide ink behind the white film resulting in improved visual compaction of the ink compared to conventional electrowetting or electrofluidic technology ( Fig. 6a ) [4] , [12] . Furthermore, the pixel borders in an electrowetting display can take up a sizeable portion of the pixel (needed to prevent ink merging, a problem the electrofluidic film eliminates). Presented in the table of Fig. 6b are theoretical optical losses, measured results and a future optimized performance. The electrofluidic film has potential to provide paper-like black/white operation ( R >76%), and with an RGBW colour filter [1] could display colour with reflectance as good as monochrome e-Ink ( R ∼ 40%) with much faster switching speed. Reflectance can be further boosted by gain reflectors [1] , which can be easily integrated onto the polymer film using microreplication. In the table of Fig. 7b , the spacers are listed as ‘not applicable’ for this work because they are clear and do not cause a loss in white reflectance. They will, however, reduce the black state and be the limiting factor for contrast ratio, because with an ink containing carbon black the rest of the display area would easily exhibit near zero-reflection (specular excluded). The spacers are typically formed with a 2:1 height:width aspect ratio. When a spacer is surrounded by ink (black state) much of the light scattered from the underlying white film will absorb at the ink touching the sidewalls of the spacer. If the spacers comprise 5% of the visual area, and as discussed above reflect only 50% of incident light in the black state, total black state reflectance (specular-excluded) would only be <3%, easily providing >30:1 contrast ratio. 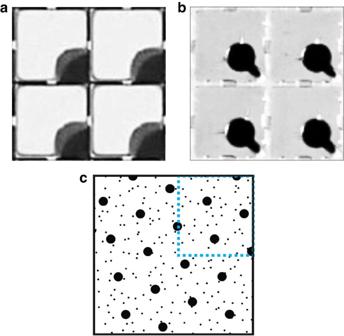Figure 7: Examples of the white state mode of the most closely related technologies. The pixels are shown in what could be a 4-pixel monochrome configuration or a 1-pixel colour configuration using an RGBW colour-filter approach and are shown to communicate the difference in reflective area for each technology. (a) An example of electrowetting display manufactured by Samsung/Liquavista14. (b) An example of a electrofluidic display developed by our working group13. (c) A diagram of the white state reflective area in an optimized electrofluidic imaging film (future work). Figure 7: Examples of the white state mode of the most closely related technologies. The pixels are shown in what could be a 4-pixel monochrome configuration or a 1-pixel colour configuration using an RGBW colour-filter approach and are shown to communicate the difference in reflective area for each technology. ( a ) An example of electrowetting display manufactured by Samsung/Liquavista [14] . ( b ) An example of a electrofluidic display developed by our working group [13] . ( c ) A diagram of the white state reflective area in an optimized electrofluidic imaging film (future work). Full size image In conclusion, a paper-like display has been created using a white porous film through which ink and clear oil fluids can be electrically transported. The sophisticated film includes numerous microfluidic design requirements, all of which have been verified experimentally. The film was also assembled without alignment to the control electrodes, a first for electrowetting or electrofluidic displays. Although this is an early stage work, both switching speed and reflectance are highly compelling, especially when compared with the existing commercial approaches based on electrophoretic or liquid crystal technologies. Low resolution 25 PPI film Figure 1 illustrates the features of the film. To fabricate the films, polycarbonate, polyethylene terephthalate and polyimide, ion track etched membranes were purchased from a commercial source (AR Brown, US) with predefined oil pore sizes from 1 and 20 μm diameters. For low-resolution films, the ink pores were defined using laser milling. The films were then coated with 100 nm of Al to serve as a grounding electrode to the polar fluid and a reflector. Some of the films are translucent, and using the Al on the backside created a diffuse white reflector. The films were dip coated with Asahi Cytop 809M to create a <100-nm hydrophobic fluoropolymer coating, providing a Young’s angle of 180° for the ink/oil combination used. High resolution 150 PPI film The same ion track etched membranes were used as discussed above; however, the definition of the ink pores was accomplished using reactive ion etching. First, a 100-nm Al coating is sputtered onto the membrane. The Al is then patterned with a wet chemical etch through a positive photoresist mask of Microposit S1818 (Shipley Company). The membranes were then dry etched 80:20 O 2 :CF 4 plasma (March CS-1507). The films were then fluoropolymer coated as described above. Even simpler methods for high-resolution film fabrication have been demonstrated, but will be reported in future publications. Electrowetting/spacer plates Indium tin oxide coated glass slides were patterned with a 36% HCl acid etch. Spacer layers of heights from 8 to 50 μm were fabricated by photolithography of SU-8 photoresist (Microchem) or PerMX 3,000 series dry film photoresist (Dupont). A dielectric layer of 0.3 to 1 μm of parylene was then coated over the electrodes and spacers. The plates were then further coated with the fluoropolymer. Fluid dosing Devices were filled with low viscosity silicone oils (Dow Chemical) and proprietary inks (pigment dispersions, Sun Chemical). First, the silicone oil was dropped onto the patterned top plate. The membrane layer was then placed on top of the oil and wicked onto the top-plate by capillary forces. The ink was then pipetted onto the exposed surface of the membrane. Last, the bottom electrode plate was brought down on top of the ink droplet to spread it over the surface. Reflection measurements An integration sphere setup used to determine percent reflection has been described in previous literature [10] . The setup is able to capture the reflectance spectrum 9° off angle with or without the inclusion of specular reflectance. Before every measurement, the setup is calibrated to a 99% diffuse white standard (Lab Sphere) ( Table 1 ). Table 1 Table comparing optical losses and net reflectance. Full size table Imaging, processing and measurement Operation was captured using CCDs. Video of device operation was taken with a DSLR camera with a 135-mm lens (Canon). For speed measurements, a high speed camera (Fastech) was used to take video at 1,000 frames per second. Video was analysed using ImageJ software. Switching times were measured by converting the video to binary mode and measuring the percentage area covered by ink versus time. The switch-on time was measured from when the ink covered 10% greater than its minimum area to 90% less than its maximum area. The reverse was used to measure the switch-off time and the two values were averaged to determine switching time. How to cite this article: Hagedon, M. et al. Bright e-Paper by transport of ink through a white electrofluidic imaging film. Nat. Commun. 3:1173 doi: 10.1038/ncomms2175 (2012).